Furrows in the wake of propagating d-cones A crumpled sheet of paper displays an intricate pattern of creases and point-like singular structures, termed d-cones. It is typically assumed that elongated creases form when ridges connecting two d-cones fold beyond the material yielding threshold, and scarring is thus a by-product of the folding dynamics that seek to minimize elastic energy. Here we show that rather than merely being the consequence of folding, plasticity can act as its instigator. We introduce and characterize a different type of crease that is inherently plastic and is formed by the propagation of a single point defect. When a pre-existing d-cone is strained beyond a certain threshold, the singular structure at its apex sharpens abruptly. The resulting focusing of strains yields the material just ahead of the singularity, allowing it to propagate, leaving a furrow-like scar in its wake. We suggest an intuitive fracture analogue to explain the creation of furrows. When handling a large sheet of paper, one must take special care not to impose boundary conditions that will result in local strains that yield the material and leave permanent defects. In fact, keeping a large sheet of paper smooth is a difficult task; more often than not wrinkles and scars appear on the surface of the paper. An example for this may be found in the mesmerizing network of scars that decorate the face of a sheet of paper after it has been crumpled to a ball and then opened [1] . In recent years, crumpled paper has attracted much attention in the scientific community and has been investigated analytically [2] , [3] , numerically [4] , [5] and experimentally [6] , [7] , [8] , [9] . In thin elastic sheets, bending deformations are energetically favourable compared with stretching deformations. Thus, a thin elastic sheet will preferentially bend to accommodate its prescribed boundary conditions and whenever possible will exhibit very little, if any, in-plane stretching. In many cases, however, the prescribed boundary conditions allow no such stretch-free configuration with finite bending energy; such is the case when a thin sheet is confined to a small volume [10] . In this case the unavoidable in-plane stretching localizes to point-like and line-like structures termed d-cones and stretching ridges, respectively [1] , [3] , [8] , [11] , [12] , [13] , [14] . It is believed that the crumpled configuration of a highly confined thin sheet can be fully described using only these two deformation modes. To determine the geometry of these singular structures, the energetic cost of in-plane stretching is balanced against the otherwise diverging bending energy. This approach has been very successful and accurately predicts the spatial structure of an isolated d-cone [11] , [15] and of a single stretching ridge [3] . The purely elastic considerations used to explain d-cone and ridge structures overlook the significant role that the time evolution of plastic deformations may have in determining the final geometry and statistics of the network [4] . One successful recent approach incorporates plasticity through the mechanism of hierarchical ridge breaking [6] , [16] , [17] . In this framework, existing defects are considered immobile and the force resisting further crumpling is associated with the nucleation of new point defects and ridges [18] , [19] . In contrast, for purely elastic sheets, point defects and their connecting ridges continuously respond to loading by the redistribution of the elastic energy through defect migration [20] , analogous to the role played by dislocations in an ordered solid. However, most materials are neither purely elastic nor fully plastic. An elastoplastic material will not only nucleate new defects in response to loading but will also allow pre-existing defects to move, leaving scars in their wake. Thus, the crumpling of elastoplastic materials is expected to exhibit highly nontrivial dissipative dynamics. Direct observation of a sheet of paper being crumpled reveals the crucial role that plasticity takes in the crumpling process, as shown in the sequence of images of a paper cylinder uniaxially compressed in Fig. 1a–d . Initially, the cylinder buckles and d-cones are created on the surface ( Fig. 1a ). Under further compression, these defects start to propagate ( Fig. 1b ) leaving a permanent elongated scar in their wake ( Fig. 1c,d ). The full dynamics of d-cone propagation and scarring on the paper have previously been observed in a cylindrical panel subjected to axial compression [21] and are also presented in Supplementary Movie 1 . The following dynamics are strongly affected by the propensity to bend along the weakened scars; thus, in addition to the traditionally considered, straight ridges connecting at vertices, the crumpled sheet is also decorated by crooked, rugged scars, reminiscent of furrows in a ploughed terrain and resulting from the propagation of individual d-cones along the surface, as shown in Fig. 1e–g . 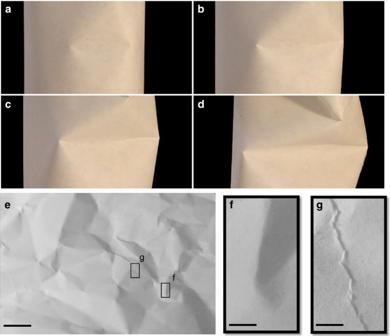Figure 1: Furrows in crumpled paper. (a–d) Furrow creation by the propagation of d-cones in a uniaxially compressed cylinder. Scale bar, 2 cm. The crease pattern of a crumpled paper, shown inewith a scale bar, 2 cm, exhibit both the classical straight ridges connecting two d-cones (f) as well as rugged furrow-like scars created by a single propagating d-cone (g). Scale bar, 2 mm. Figure 1: Furrows in crumpled paper. ( a – d ) Furrow creation by the propagation of d-cones in a uniaxially compressed cylinder. Scale bar, 2 cm. The crease pattern of a crumpled paper, shown in e with a scale bar, 2 cm, exhibit both the classical straight ridges connecting two d-cones ( f ) as well as rugged furrow-like scars created by a single propagating d-cone ( g ). Scale bar, 2 mm. Full size image To better understand this new type of creases, which are inherently plastic and are formed by the propagation of single point defects, we create and manipulate them in isolation. We observe that a single d-cone in the centre of an elastoplastic Mylar sheet will initially remain pinned in place even when force is applied to it. However, once the force reaches a critical value, F y , the d-cone sharpens abruptly; this focuses the stresses at the tip and the d-cone begins to propagate across the sheet. The force required to propagate the singularity and elongate the furrow scales quadratically with the thickness of the sheet. Experimental set-up We experimentally probe the propagation of point defects and resulting scarring in thin sheets by studying single d-cones embedded in commercial Mylar sheets. The sheets, 50–250±5 μm in thickness, are cut to circles of 45 mm in radius. To controllably form an initial d-cone, we follow the procedure described by in ref. 15 and shown in Supplementary Movie 2 . The Mylar sheet is manually pushed into a rigid ring with an inner radius of 29 mm. The pushing force is applied to the centre of the Mylar sheet perpendicular to the plane of the plastic ring, and the total penetration depth of the centre of the sheet into the plastic ring is 7.5 mm. This procedure results in the formation of a single d-cone at the centre of the Mylar sheet: a finite region supported on the plastic ring and forming a section of a cone and a free standing region concave at its centre and flanked by two convex regions. The sheet is then removed from the confining ring while retaining the d-cone structure, and transferred to a three point support, one above the sheet in the concave region, and two below the sheet in the convex regions, as shown in Fig. 2 . The geometry of the three point support, composed of 0.5′′ metal posts, is then fixed such that the central supporting post lies in the xz plane at an angle of ∼ 50° with the x axis. The supports of the flanking regions lie in the xy plane at an angle of ∼ 57° with the x axis as shown in Fig. 2 . This results in a 3D tetrahedral geometry where the imaginary continuations of all three posts meet at the d-cone, as shown schematically in Fig. 2b–d . The sheet is rigidly clamped only to the central pole. The front conical section of the sheet is initially free and unsupported. The d-cone preparation and loading procedure is shown for a typical example in Supplementary Movie 2 . 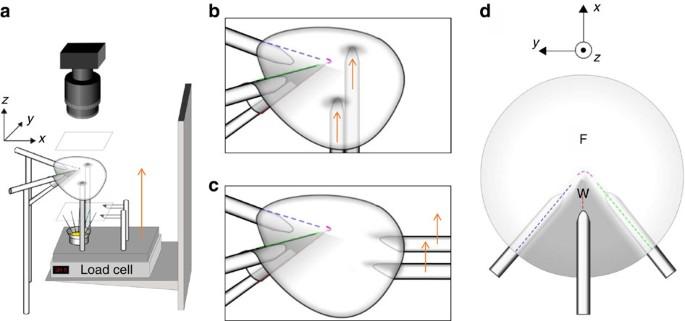Figure 2: Experimental set-up. (a) A schematic illustration of the experimental set-up. (b,c) An illustration of the two loading geometries used: vertical (b) and horizontal (c). (d) A schematic top view of the supporting posts and the sheet, indicating the front (F) and the wake (W) of the advancing d-cone. Figure 2: Experimental set-up. ( a ) A schematic illustration of the experimental set-up. ( b , c ) An illustration of the two loading geometries used: vertical ( b ) and horizontal ( c ). ( d ) A schematic top view of the supporting posts and the sheet, indicating the front (F) and the wake (W) of the advancing d-cone. Full size image To advance the d-cone, load is applied to the thin sheet by two parallel cylindrical posts that are fixed at the conical region of the d-cone at equal distances from the x axis and separated from each other by 25 mm. The posts are displaced vertically at a constant rate of 0.5 mm s −1 . The loading posts are mounted on a Sartorius TE6101 scale, and the force that the sheet exerts against them is continuously recorded at a frequency of 3.8±0.1 Hz. The scale and the loading posts are placed on a moving stage (Thorlabs LTS300) and are displaced vertically as one unit. We use two configurations of the loading posts: vertical relative to the xy plane ( Fig. 2b ), for which the contact with the sheet is constant in the xy plane and horizontal relative to the xy plane ( Fig. 2c ), where contact with the sheet is not constant in xy but remains stationary on the circumference of the sheet. For vertical loading geometry, load is applied closer to the d-cone, making the sheet less susceptible to global buckling and allowing us to probe a larger range of loads, while the horizontal loading geometry is more convenient for imaging. The deformation of the sheet is imaged in real time using photoelasticity, as described in the Methods section. Force measurements and focusing of d-cones When the loading posts move up, the Mylar sheet resists its deformation and exerts a normal force, F(z) , against the posts. F(z) has a characteristic functional form universal to all the different sheet thicknesses, h , as shown for a horizontal loading configuration in Fig. 3a . We identify two distinct regimes in the evolution of F(z) , static and dynamic, as highlighted by the two colour shadings in the inset to Fig. 3a . In the static regime, the tip of the d-cone maintains its position throughout the loading process, while F(z) increases monotonically. When the force reaches a critical value, F y , F(z) abruptly decreases as the d-cone yields and begins to propagate in the x direction. We therefore refer to this regime as dynamic. Note, however, that if the loading is halted, the d-cone arrests instantly and F(z) monotonically decays over time, as shown in the inset to Fig. 3b . Once loading is resumed, a larger force is necessary for the d-cone to re-initiate motion, as shown in Fig. 3b . The decrease in the force following F y is concomitant with the dynamic propagation of the d-cone and marks the transition from the static to the dynamic regime, as shown in Supplementary Movie 3 . In the dynamic regime, F(z) remains nearly constant and scales as h 2 . This is shown by the collapse of the curves following the yield event in Fig. 3c . For vertical loading geometry, the behaviour is qualitatively similar, as shown in Fig. 3d . However, in this geometry the force propagating the d-cone increases monotonically with z . This is due to the decreasing distance between the propagating d-cone and the loading points, which in this loading geometry are fixed in the xy plane. As the distance between the d-cone and the loading posts diminishes, the torque is applied to the d-cone over a shorter leverage and thus decreases. Nevertheless, F(z) scales as h 2 for the vertical loading geometry as well, despite the difference in its functional form, as shown in the insets to Fig. 3d . Within the static regime, F(z) does not exhibit any simple scaling with h . Nevertheless, the rise of F(z) to its critical value and the transition into the plastic regime occurs considerably more abruptly for thinner sheets. 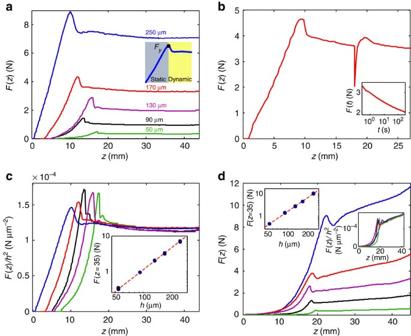Figure 3: Force measurements. (a)F(z)for different thicknesses,h, under horizontal loading geometry. (Inset)Fyseparates between the static and dynamic regimes. (b)F(z)for a 170-μm-thick sheet. Atz=18 mm the loading posts are stopped and held in place for 300 s before increasing ofzis resumed. (Inset)F(t)as a function of time passed since stopping the loading posts. (c)F(z)normalized byh2. (Inset)F(z=35) as a function ofh. The red line of slope two is added as a guide to the eye. (d)F(z)for vertical loading geometry. (Insets)F(z)normalized byh2andF(z=35) as a function ofh. Figure 3: Force measurements. ( a ) F(z) for different thicknesses, h , under horizontal loading geometry. (Inset) F y separates between the static and dynamic regimes. ( b ) F(z) for a 170-μm-thick sheet. At z =18 mm the loading posts are stopped and held in place for 300 s before increasing of z is resumed. (Inset) F(t) as a function of time passed since stopping the loading posts. ( c ) F(z) normalized by h 2 . (Inset) F(z =35) as a function of h . The red line of slope two is added as a guide to the eye. ( d ) F(z) for vertical loading geometry. (Insets) F(z) normalized by h 2 and F(z =35) as a function of h . Full size image For the d-cone motion to initiate, the core structure of the d-cone must undergo a geometrical transition and focus the stresses at its leading edge. This is shown clearly in the dramatic sharpening of the d-cone shown in Fig. 4a between z =5 and z=10 mm, and additionally in the corresponding Supplementary Movie 3 . In the static regime, external loading is accommodated by large-scale deformation over the length of the entire sheet, while the shape and location of the d-cone remain practically unaffected, as shown for z =0 and z =5 in Fig. 4a,b . Then, when loading force reaches F y , the radius of the d-cone crescent-shaped core, r c , sharply decreases and the singularity starts to propagate, with no further significant change in r c . The abrupt focusing of r c occurs simultaneously with the drop of F(z) , as shown in Fig. 4b and in Supplementary Movie 3 . r c scales approximately linearly with the sheet thickness in both the static and dynamic regimes; however, within the dynamic regime the d-cone is approximately sevenfold sharper, as shown in Fig. 4c . 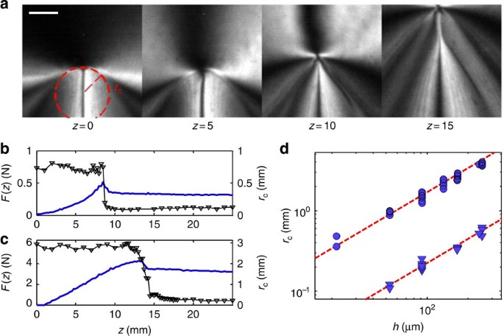Figure 4: Propagation of the singular structure is preceded by the focusing of stresses at the tip. (a) Four typical snapshots showing a 50-μm-thick sheet placed between two crossed linear polarizers at four different values ofz. Scale bar, 1 mm. (b,c)rc(z)(black triangles) andF(z)(blue line) as a function ofzforh=50 μm (b) andh=170 μm (c) under horizontal loading geometry (d)rcversushin the static regime (circles) and dynamic regime (triangles). The two red lines of slope one are added as guides to the eye. Figure 4: Propagation of the singular structure is preceded by the focusing of stresses at the tip. ( a ) Four typical snapshots showing a 50-μm-thick sheet placed between two crossed linear polarizers at four different values of z . Scale bar, 1 mm. ( b , c ) r c (z) (black triangles) and F(z) (blue line) as a function of z for h =50 μm ( b ) and h =170 μm ( c ) under horizontal loading geometry ( d ) r c versus h in the static regime (circles) and dynamic regime (triangles). The two red lines of slope one are added as guides to the eye. Full size image The linear scaling of r c observed in Fig. 4c , while obtained over a range of only one decade, cannot be reconciled with the scaling of r c ∼ h 1/3 previously obtained for d-cones in purely elastic sheets [11] , [22] . In these experiments and simulations, the d-cone is formed by pushing a thin disc at its centre through an impenetrable ring. This results in a buckled shape whose angular opening is unconstrained and is determined by bending energy minimization alone. Following this highly symmetric loading protocol, we are indeed able to recover the r c ∼ h 1/3 scaling result (see Supplementary Fig. 1 ). However, once the buckled shape is further loaded and constrained, as one may expect to occur in real crumpled sheets, we observe the linear scaling. In the dynamic regime the loading force obeys the scaling relation F(z,h)=F(z) × h 2 for both loading geometries, as shown in Fig. 3c and the insets to Fig. 3d . This scaling can now be understood by examining the cross-sectional area of the irreversibly deformed region, and using the linear dependence of r c on the thickness of the sheet. We balance the work done by F(z) with the dissipation associated with creating a furrow at the wake of the propagating d-cone. The d-cone focuses the deformation to a region of width r c ∼ h , giving rise to furrows of similar width. This irreversible deformation occurs throughout a finite fraction of the thickness of the sheet, h ; consequently, this results in a dissipation rate that is proportional to h 2 , consistent with our measurements. This simple scaling argument suggests a propagation criterion for a d-cone that is analogous with the energy balance used to describe crack propagation in fracture mechanics. Similar experiments were made for different materials to check the universality of the scaling behaviour (see Supplementary Fig. 2 and Supplementary Table 1 ). Although measurements for materials such as paper are noisier, they are consistent with the h 2 behaviour and observed across different materials—plastics, papers and metals. The h 2 scaling will also be typical for the critical torque needed to form a plastic hinge [23] , thus suggesting that the plastic scarring results solely from localized bending deformations. However, identical scaling could also be obtained for in-plane stretching by accounting for the length scale over which plastic flow occurs (see Discussion). Consequently, our results cannot rule out the role of in-plane stresses in the plastic deformation. It is important to note that the above argument does not imply that a furrow will form and propagate as soon as the force-dissipation balance is met. In order to generate a furrow from a simple d-cone at rest, additional focusing must take place, as observed in Fig. 4 . The threshold force for this focusing, F y , scales similarly with the thickness, but tends to be higher than the force needed to advance a furrow. In the static regime, the d-cone shape is blunt and the load is distributed over a wide region, allowing the tip to persist under high loads before yielding. When the yield force is reached the d-cone tip sharpens, thus significantly focusing the applied load to a small region in which the plastic deformation takes place. The tip of the d-cone remains sharp throughout the dynamic regime, localizing deformations more effectively and requiring less force in order to set the d-cone in motion. Dependence of yield force on the d-cone size The focusing of stresses at the tip of the d-cone is analogous to the parabolic displacement profile of a crack, where the singular profile of the crack effectively focusses elastic stress and all of the plastic dissipation is localized to a small process zone at the tip of the crack. A common method to stop or delay crack propagation in brittle solids is to blunt their stress-focusing mechanism. This is accomplished by rounding the otherwise sharp crack tip. We achieve the same goal for d-cones by using laser engraving to introduce well-defined initial crescent-shaped scars on the Mylar sheets. The crescent scars are weak lines for bending deformations and serve to guide the formation of the d-cones around a chosen core in the shape of a circular arc of radius r 0 . The shape of the supported thin sheet away from the scar remains unaltered; nevertheless, in the vicinity of the scar the deformation of the core is significantly different than that of the generic d-cone, as shown in Fig. 5a . We repeat the vertical loading experiments with the laser-engraved Mylar sheets for radii r 0 ranging from 1 to 20 mm and find that the functional form of F(z) in the static regime is insensitive to r 0 ; however, regions of higher initial curvature focus stresses more efficiently, resulting in lower values of F y for smaller r 0 values, as shown in Fig. 5b . The decrease in the force accompanying the onset of propagation is more abrupt for the artificial scars than for the ordinary d-cone. However, once the d-cone propagates away from the initial engraved scar, F(z) is again independent of r 0 , and all curves converge to one. For a given sheet thickness, F y scales as F y ∼ r 0 1/3 , as shown in the inset to Fig. 5c . In addition, when F y is rescaled by h 2 and plotted as a function of r 0 /h , all the data collapse on a universal master curve, as shown in Fig. 5c , suggesting the following scaling for the critical force: F y (h,r 0 ) ∼ h 5/3 r 0 1/3 . 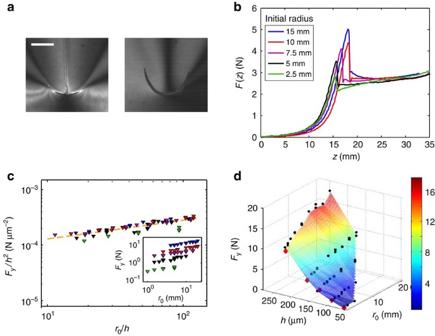Figure 5: Imprinted crescent scars as d-cone surrogates. (a) Images of a Mylar sheet with a generic d-cone (left) and a laser-engraved crescent defect (right) mounted on the supporting posts and imaged between two crossed polarizers. Scale bar, 1 mm. (b)F(z)forh=130 μm with varying initial radii,r0. (c)Fy/h2as a function ofr0/hfor differenth, colour-coded as in previous figures. The orange line of slope 1/3 is added as a guide to the eye. (Inset)Fyas a function ofr0for differenth. (d) Three-dimensional plot ofFyas a function ofr0andh. The surfaceFy(h,r0) is interpolated numerically from the yield force values measured for the laser-engraved sheets (black dots). The red diamonds correspond to the average values ofFy(h)measurement on generic d-cones. Figure 5: Imprinted crescent scars as d-cone surrogates. ( a ) Images of a Mylar sheet with a generic d-cone (left) and a laser-engraved crescent defect (right) mounted on the supporting posts and imaged between two crossed polarizers. Scale bar, 1 mm. ( b ) F(z) for h =130 μm with varying initial radii, r 0 . ( c ) F y /h 2 as a function of r 0 /h for different h , colour-coded as in previous figures. The orange line of slope 1/3 is added as a guide to the eye. (Inset) F y as a function of r 0 for different h . ( d ) Three-dimensional plot of F y as a function of r 0 and h . The surface F y (h,r 0 ) is interpolated numerically from the yield force values measured for the laser-engraved sheets (black dots). The red diamonds correspond to the average values of F y (h) measurement on generic d-cones. Full size image Despite the differences between the standard d-cone geometry and d-cone around the artificial scar, the value of the yield force, F y (h,r 0 ), approaches the generic d-cone value, F y , as r 0 approaches r c from above, as indicated by the full red diamonds in Fig. 5d . Values of r 0 below r c were experimentally inaccessible; bellow a critical radius the sheet could not be manually forced into a d-cone-like geometry around the smaller crescent scar. Interestingly, these minimal values of r 0 are very close to the initial r c values of the d-cone created by pushing a sheet through a ring. Yet, in spite of this apparent lower bound to the scale over which deformation can initially occur, it is surprising to note that after yielding the tip focuses further by nearly an order of magnitude. Further studies are required to identify the exact mechanism for the focusing of the d-cone and its scaling. To fully understand the role that plasticity plays in the dynamics of crumpling, we must consider the mechanism underlining the dynamics of furrow creation. The first critical step for this is the distinction between yielding due to bending and to that resulting from stretching. For a d-cone core of spatial dimensions that scale linearly with the thickness, h , we expect a maximal Gaussian curvature that scales as h −2 , leading to a maximal in-plane strain that is independent of the thickness through ɛ ∼ ∇ −2 K ∝ O (1). The linear core scaling also implies a maximal curvature that scales as k max ∼ h −1 and consequently a curvature-induced maximal strain, k max h , that is independent of the thickness. Thus, in-plane-strain-induced deformations and curvature-induced deformations both give rise to maximal strains that do not depend on the thickness and could be the source of plastic yield. Moreover, accounting for the length along which we expect the yield stress to be achieved we obtain for in-plane-stress induced yielding F ∼ σ Y h 2 , which is also consistent with the measured scaling. Thus, on the basis of the evidence we presently have we cannot completely dismiss the role of in-plane stretching in the plastic deformation process. Nevertheless, it is not unlikely that such stresses play a crucial role in the pinning of the d-cone and facilitate the sharpening of the tip of the d-cone, allowing it to propagate across the thin sheet. Imaging using photoelasticity The deformation of the sheet is imaged in real time with a digital camera (Thorlabs DCC1545M CMOS) positioned directly above it. We use photoelasticity to highlight the deformation; the Mylar sheet is illuminated with a white LED from bellow and placed between two crossed linear polarizers. The Mylar sheets are anisotropic and display linear birefringence at zero strains; thus, in addition to the photoelastic effect, the polarization of light transmitted through the Mylar sheet is influenced by the relative orientation of the Mylar sheet with respect to the orientation of the polarizers, and with respect to the direction of light propagation. How to cite this article: Gottesman, O. et al . Furrows in the wake of propagating d-cones. Nat. Commun. 6:7232 doi: 10.1038/ncomms8232 (2015).